Topological excitations in a kagome magnet Chirality—that is, left or right handedness—is present in many scientific areas, and particularly in condensed matter physics. Inversion symmetry breaking relates chirality with skyrmions, which are protected field configurations with particle-like and topological properties. Here we show that a kagome magnet, with Heisenberg and Dzyaloshinskii–Moriya interactions, causes non-trivial topological and chiral magnetic properties. We also find that under special circumstances, skyrmions emerge as excitations, having stability even at room temperature. Chiral magnonic edge states of a kagome magnet offer, in addition, a promising way to create, control and manipulate skyrmions. This has potential for applications in spintronics, that is, for information storage or as logic devices. Collisions between these particle-like excitations are found to be elastic at very low temperature in the skyrmion-skyrmion channel, albeit without mass-conservation. Skyrmion–antiskyrmion collisions are found to be more complex, where annihilation and creation of these objects have a distinct non-local nature. Systematic studies of strongly interacting electronic systems had been based on the formalism of Landau Fermi liquid for a long time. Landau pointed out that a strongly correlated problem can be replaced by a set of quasiparticles and effective amplitudes describing the interaction among them. Each quasiparticle is characterized by its own effective mass and can be adiabatically connected to a weakly interacting Fermi gas. A proper many-body description of solid-state systems cannot be addressed within linear theory; however, small anharmonic perturbations do not change qualitatively the quasiparticle picture and can be treated as scattering processes between them, leading to multiple harmonic generation, quasiparticles dressing, and so on [1] . The inability to explain a variety of phenomena within perturbative expansions have motivated the development of novel mathematical concepts. Since the second half of the twentieth century, topological methods have played an increasingly important role in different branches of physics owing to their utility in analysis of high-complexity field equations that do not allow a simple general solution. The quantum Hall effect [2] , Aharanov–Bohm’s effect [3] and the Josephson junction [4] are some examples in which topological arguments help to elucidate the physical origin of the observed phenomena. A certain class of nonlinear equations allows particle-like solutions, solitary waves or solitons. Thus, a soliton, a freely moving self-trapped state of a nonlinear system, can be thought of as a clot of energy concentrated in a small area that is able to move while preserving its shape. Contrary to ‘true’ solitons that preserve their shape during and after collision, there exists so-called topological solitons (soliton in a broader sense) that are characterized by a non-trivial topological entity—topological charge. These particular solitons are known as topological excitations since their stability purely relies on topological arguments and cannot be adiabatically connected to their ground states. The topological excitations are basically determined by the dimension of the space and the order parameter. Thus, for example, in a two-dimensional (2D) space, a Heisenberg ferromagnet allows an excitation called the Belavin–Polyakov monopole [5] . For this particular example, the Belavin–Polyakov excitation is equivalent to a skyrmionic particle-like solution [6] because of the conformal invariance of the Heisenberg Hamiltonian in two dimensions. In what follows we focus our attention on a skyrmion, a topological soliton corresponding to a nonlinear σ model. The concept of the skyrmion originates from the seminal work of Skyrme [6] who argued that a topologically protected field configuration in a continuous field has particle-like solutions (that is, skyrmions). A pioneering use of the Skyrme model was employed to describe stable elongated particles (baryons) within the framework of nonlinear theory of meson fields. The model is characterized by a conserved baryon number, a topological charge, which is independent of the equations of motion and allows to develop a theory of nucleons obeying a mesonic Fermi statistic (Bose fields) [7] . Within the theory in question, the baryon is nothing but a chiral soliton resulting in collective excitations of pion fields. Its appearance can be attributed to spontaneous breaking of chiral symmetry, while the model itself reveals the nature of Fermi—Bose transmutation. Thanks to that, the skyrmion became known as a particle-like solution in purely bosonic theories obeying Fermi statistics. Developing this idea introduced a new class of particles with fractional statistics, anyons, which are now widely used. Skyrme’s proposal has been extended beyond the scope of high-energy physics and in material science has been an important concept in new and exotic physics, for example, in nematic liquid crystals [8] , ferromagnetic Bose–Einstein condensates [9] , high T c superconductivity [10] and quantum Hall magnets [11] . Studying low-dimensional magnetic structures remains one of the most challenging and fascinating fields of modern condensed matter physics. Depending on the distance between neighbouring spins, crystalline symmetry and hybridization with substrate, a wide range of magnetic configurations ranging from collinear ferromagnetic, antiferromagnetic and non-collinear helimagnetic configurations to more complicated textures can be observed. If, in addition, the inversion symmetry of the system is broken, the spin alignment/configuration gains a certain chirality (handedness) because of the spin–orbit (SO)-driven antisymmetric exchange interaction, that is, Dzyaloshinskii–Moriya (DM) interaction. Magnetic skyrmions are chiral spin structures with a whirling configuration so that the plane on which the spins are specified is topologically equivalent to a sphere via, for example, a stereographic mapping. Because of that a certain topological invariant namely degree of mapping can be ascribed to the structure. It can be thought of as a skyrmion number as well, providing information analogous to the charge in a particle-like description. One can also evaluate the accumulated Berry phase that influences, for example, travelling electrons when they pass through a skyrmion [12] . Recently, it has been shown that the Berry phase gives rise to the DM interaction in the case of smooth magnetic textures when both inversion symmetry is broken and SO interaction is present [13] . We argue in this communication that the aforementioned intrinsic property makes a kagome ferromagnet ideal for creating and controlling the movement of skyrmions. From a technological perspective, skyrmions are promising objects because of their stability. This comes about from the topological nature of the skyrmion, which prevents a continuous deformation into another magnetic configuration with a different topological invariant. Indeed, the existence of topological invariance originates in the duality between - and -space and, as a consequence, when dealing with the group velocity, its standard quasiclassical expression gains an anomalous term, which is proportional to the so-called Berry curvature. Mathematically, the integral of the Berry curvature over a 2D manifold defines an integer invariant, a first Chern class [14] . For a system that is time-reversal invariant and spatial-inversion invariant, the Berry curvature vanishes. Thus, the Chern number is zero unless the symmetry is broken. In 2D systems, the bands with non-zero Chern numbers must be separated from the other bands by a band gap, such that the boundary between topological phases with different Chern numbers (or other topological invariants) must support the edge modes (similar to the electronic structure at the surface of a topological insulator). Because of the aforementioned properties, the skyrmions are appealing for applications in information storage or logic devices. However, they need to meet several requirements in order to be useful for magnetic applications, namely, they need to have high mobility, small size and should allow for full control of the direction of movement. In this article, we report on the conditions under which skyrmions are created in a kagome lattice, and we show that this system has all the aforementioned technologically relevant properties. Topological bulk and edge states The vanadate pyrochlores with generic formula A 2 V 2 O 7 (A=Lu, Yb, Tm, Y) form a class of ferromagnetic insulators, where the V atoms carry a magnetic moment of ~1.0 μ B per atom. A very important member of this family is Lu 2 V 2 O 7 , in which very recently the magnon Hall effect has been observed [15] and in addition it was predicted to be a topological magnon insulator [16] . In this compound only V atoms carry a magnetic moment, since Lu is trivalent with a filled 4f shell. The structure of this vanadate (the unit cell is displayed in Fig. 1a ) can be represented as a stacking of alternating kagome and triangular lattices along the [111] direction. In Fig. 1b , we show the stacking of these layers, in such a way that inversion symmetry is broken. As a consequence, the DM interaction is non-zero. According to Moriya’s rules [17] on a single tetrahedron, the DM vector on each bond is parallel to the surface of the surrounding cube and perpendicular to the bond as indicated in Fig. 1c with blue arrows. We concentrate here our efforts on a model system given by a ferromagnetic kagome lattice as shown in Fig. 1d for vanadium atoms of Lu 2 V 2 O 7 . The relevant factor in our analysis of topological excitations in the kagome magnet is represented by the ratio between the antisymmetric ( ) and isotropic ( ) exchange interactions, namely . This ratio captures the basic features about the interactions present in the Lu 2 V 2 O 7 pyrochloride. In experiments [15] , has been found to be close to 0.32. Our simulations, described in the Methods section, show that the creation and manipulation of skyrmions in the kagome lattice do not rely too much on small variations of this ratio. Hence, although our results, shown below, are for , our theoretical predictions at 1 mK are expected to be relevant for the V atoms forming a kagome lattice in the pyrochloride Lu 2 V 2 O 7 as well as systems with similar ratio. 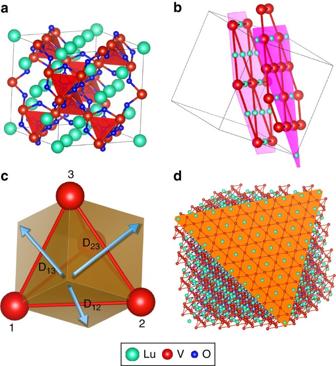Figure 1: Crystal structure of Lu2V2O7. (a) Pyrochlore structure of Lu2V2O7. (b) Graphical representation of the alternating stacking of triangular and kagome layers of the pyrochlore lattice. (c) Schematic representation of the Dzyaloshinskii–Moriya vector for the atoms that form the plane of the kagome lattice. (d) Vanadium kagome lattice as a result of cutting a surface-plane perpendicular to the direction [111]. Notice that the colour coding of the different type of atoms is the same ina–d. Figure 1: Crystal structure of Lu 2 V 2 O 7 . ( a ) Pyrochlore structure of Lu 2 V 2 O 7 . ( b ) Graphical representation of the alternating stacking of triangular and kagome layers of the pyrochlore lattice. ( c ) Schematic representation of the Dzyaloshinskii–Moriya vector for the atoms that form the plane of the kagome lattice. ( d ) Vanadium kagome lattice as a result of cutting a surface-plane perpendicular to the direction [111]. Notice that the colour coding of the different type of atoms is the same in a – d . Full size image In a kagome ferromagnet (described by a Hamiltonian, as given in equation (1)), the DM interaction is not forbidden by the symmetry of the lattice because the middle point between two sites is not an inversion centre. Consequently, in the presence of significantly large DM interactions, the magnon dispersion curves of a kagome magnet present similarities with the energy band spectra of topological insulators. In fact, in such a system the magnon dispersion relation is gapped in the bulk but allows travelling gapless edge states that are topologically protected against any variation of the material parameters unless the band gap in the bulk collapses. Even though our studied sample is one-atomic-layer thick system, we denote hereafter bulk states by the states that exist well inside the sample and consequently, by abuse of language bulk skyrmions, refers also to the skyrmions that exist inside the 2D sample. We consider here magnetic excitations of a 2D kagome lattice, for example, as given by a [111] surface of the pyrochlore lattice (see Fig. 1d ) at a temperature of 1 mK, unless stated otherwise. We assume a very low temperature in the majority of our simulations because the results described here are easier to observe at that temperature, and most likely also in experiments, because the perturbations from thermal fluctuations are smaller. Very low temperature conditions make the analysis easier; however, we have also analysed the conditions to stabilize skyrmions at room temperature in the penultimate subsection. We start by analysing bulk and edge states of this system, and to this end we show in Fig. 2a the magnon dispersion, as revealed from the dynamical structure factor. Note that the results in Fig. 2a are obtained using open boundary conditions for a large sample composed of 50 × 400 unit cells. The intense coloured curves represent bulk magnons, which are seen to be grouped in three branches, with noticeable gaps in-between. Most noteworthy is that in between the gaps one can find four twisted edge states that form a continuous state. These states cannot be perturbed, so that a gap opens because they represent edge modes that are topologically protected. In fact, the presence of a DM interaction with a fixed handedness acts as an effective magnetic field in the system (see Supplementary Note 2 ). This makes the magnon spectrum of the kagome lattice looks similar to the energy band structure of topological insulators. Similar magnon dispersion relations have been calculated in ref. 16 using a model hamiltonian as described in equation (1). In ref. 16 , the properties related to the nondissipatively heat transport by the magnons were studied. In the present work, we are focused on the generation and manipulation of topological excitations as well as their collisions. In order to analyse the edge and bulk modes in real space, we show the real-space Berry curvature, averaged over a time interval of 100 ps, in Fig. 2b,c (see Supplementary Note 1 for further details about the calculation of the Berry curvature and topological invariants in the framework of our theoretical method). The results of Fig. 2b,c were obtained after exciting the first two rows of atoms with an external magnetic field on the left side of the sample, and then the time evolution of the system was monitored. The excitation was carried out first with an energy of 261 meV and second with an energy of 814 meV. The first excitation represents magnon energies that are allowed in the bulk, whereas the second excitation represents an energy for which bulk states are forbidden, since this energy lies in the magnon gap. 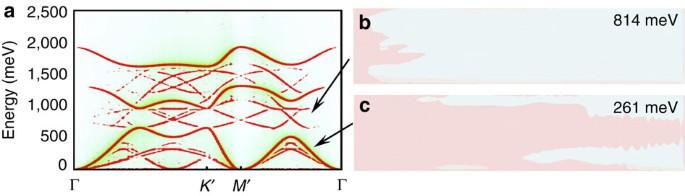Figure 2: Topological magnonic bulk and edge states in a kagome lattice. (a) The dynamic structure factor is shown along the high symmetry points Γ→K′→M′→Γ, whereK′=2KandM′=2M.K′andM′are referred to as points in the extended Brillouin zone. (b,c) Berry curvature shown in real spin-space averaged over a time interval of 100 ps (seeSupplementary Note 1). Inb,c, the system is perturbed with an energy of 814 and 261 meV, respectively. Moreover, theratio has been chosen to be 0.4 and T=1 mK. The red colour indicates an excitation where the atomic magnetic moment deviates from the ground-state orientation that is represented by the moments pointing almost along thezaxis. Blue-light colour represents atomic moments oriented almost along thezaxis in a ground-state configuration. Figure 2c (261 meV case) displays spin waves that propagate over the whole sample, corresponding to the expected bulk modes of the 261-meV excitation, whereas Fig. 2b (814 meV case) shows magnon excitations that only propagate along the edges, that is, representing edge modes. The data in Fig. 2a–c demonstrate that magnetic excitations of a kagome lattice have just as rich physics, in terms of non-trivial topology, as the electronic structure of topological insulators. The advantage with investigations of magnetic excitations is that it is possible to keep track of the real-space information of the magnetic excitation as a function of time, for example, as given by the information in Fig. 2b,c . Figure 2: Topological magnonic bulk and edge states in a kagome lattice. ( a ) The dynamic structure factor is shown along the high symmetry points Γ→ K ′ → M ′ →Γ, where K ′ =2 K and M ′ =2 M . K ′ and M ′ are referred to as points in the extended Brillouin zone. ( b , c ) Berry curvature shown in real spin-space averaged over a time interval of 100 ps (see Supplementary Note 1 ). In b , c , the system is perturbed with an energy of 814 and 261 meV, respectively. Moreover, the ratio has been chosen to be 0.4 and T=1 mK. The red colour indicates an excitation where the atomic magnetic moment deviates from the ground-state orientation that is represented by the moments pointing almost along the z axis. Blue-light colour represents atomic moments oriented almost along the z axis in a ground-state configuration. Full size image Local topological excitations Next, we consider local excitations, for example, as they would emerge from a spin-transfer torque of a spin-polarized scanning tunnelling microscope tip or as described in the experiments of ref. 18 . This excitation was generated by applying a local torque that causes all the atomic spins subjected to this torque to have their moments reversed with respect to the majority of the spins in the simulation cell ( Fig. 3 shows the configuration at t =0 ps). We then removed this torque and observed that the remaining excited state is similar to a skyrmion-like or a skyrmion–antiskyrmion (SA) pair, which in most simulations were stable for long times (>100 ps). This procedure was repeated several times and it was found that skyrmionic excitations were always stabilized (see Supplementary Note 3 for further details about the role played by the DM interaction and the kagome lattice in the stabilization of the solitonic solutions described hereafter). Their stability is very much dependent on the damping parameter because this parameter takes care about the energy dissipation in the system (see Supplementary Note 4 ). We have found that for a damping below ~0.01, the solitonic excitations have a lifetime longer than the simulation time (≈100 ps). 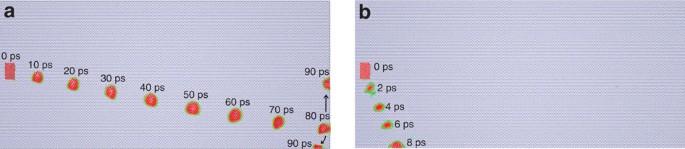Figure 3: Snapshots of two skyrmionic excitations created in the centre of the kagome stripe. (a) Time evolution of an SA pair, and the generation of a meron and antimeron after colliding with the edge of the sample. The measured SA pair speed is ~1,290 m s−1(Supplementary Movie 1). (b) Same simulation conditions as ina, but with different direction of the linear momentum of the SA pair because of the nonlinear process of the SA pair generation (see text andSupplementary Movie 2). The blue colour represents the atomic spins pointing in the out-of-plane direction, while red colour means that the magnetization is reversed 180 degrees. The green colour represents atomic spins lying in-plane. Same colour convention applies throughout the rest of this paper. In both figures, we only show the right half side of the kagome stripe so that the rectangular excitation at 0 ps is located in the centre of the stripe. The calculations were performed withT=1 mK,mRy andmRy. Figure 3 shows the generation and time evolution of two such skyrmionic excitations (a movie of these excitations is found in Supplementary Movies 1 and 2 ). It may be seen that they are both stable but that the initial direction of their movement is different (see Fig. 3a,b ). Figure 3: Snapshots of two skyrmionic excitations created in the centre of the kagome stripe. ( a ) Time evolution of an SA pair, and the generation of a meron and antimeron after colliding with the edge of the sample. The measured SA pair speed is ~1,290 m s −1 ( Supplementary Movie 1 ). ( b ) Same simulation conditions as in a , but with different direction of the linear momentum of the SA pair because of the nonlinear process of the SA pair generation (see text and Supplementary Movie 2 ). The blue colour represents the atomic spins pointing in the out-of-plane direction, while red colour means that the magnetization is reversed 180 degrees. The green colour represents atomic spins lying in-plane. Same colour convention applies throughout the rest of this paper. In both figures, we only show the right half side of the kagome stripe so that the rectangular excitation at 0 ps is located in the centre of the stripe. The calculations were performed with T =1 mK, mRy and mRy. Full size image The size and magnitude of the linear momentum of the skyrmionic excitation is in general found to be stochastic and depends on minute details of the conditions of the spin system just after removing the local torque. As discussed above, this is noticeable when comparing Fig. 3a,b . In both figures, the simulation parameters were exactly the same; however, the highly nonlinear process of the creation of the SA pair, combined with small thermal fluctuations, edge effects on the spin-reversed region at the beginning of the simulation and so on causes the direction of the linear momentum of the skyrmionic excitation to be very different. Furthermore, in Fig. 3b , the excitation is found to experience stronger damping, in a process that emits spin waves. As a result of the new direction, the SA pair collides with the edge 8 ps after it is created. The velocity of the SA pair in Fig. 3b is ~4,516 m s −1 . Therefore, the velocity is basically four times bigger than the velocity of the SA pair in Fig. 3a . Although the topological edge modes should retain the SA pair on the edge, however, as we stated above, the topological stabilization only works for small perturbations. In Fig. 3b , the velocity as well as the linear momentum are considerably large so that when the SA pair collides with the edge of the kagome magnet, the energy is so large that it cannot nonetheless be absorbed by the edge mode and the energy is released or emitted via spin waves. The results in Fig. 3 demonstrate that SA pairs are easily generated in the interior of the kagome lattice but that there is an uncertainty in the determination of their linear momentum and their lifetime. The competition between exchange and DM interaction favours canted magnetization and, as a result, the effects associated with finite size geometry are of crucial importance. A non-trivial magnetic texture is in general subjected to the Magnus force, which prevents it from moving to the boundary. However, it can be easily shown that as long as the strength of a local torque is sufficiently small, a repulsion from the edge is circumvented. In Fig. 3a , a coupled SA pair has time to become stabilized (~80 ps) and is found to travel with a speed of ~1,290 m s −1 to the right edge of the sample. The linear momentum is large enough for the SA pair to reach the edge, where it splits into a separate meron and antimeron (the meron is a topological soliton with non-integer topological charge, discussed further below). Both the meron and antimeron are stable during a significant period of time, that is, at least longer than 10 ps. The results in Fig. 3 motivate an analysis in terms of a meron [19] (in our case, half-skyrmion) that originally was introduced to resolve the problem of confinement in particle physics, namely when quarks are bound by strong forces at large distances [20] . The latter fact prevents the application of a semiclassical approximation directly. In fact, within the semiclassical approach one may look for a perturbative expansion around the minima of the Euclidean action (this effectively leads to a series obtained by re-summing an infinite number of graphs). Thus, using this formalism restricts one to finite-action solutions, also known as instantons. However, elevated temperatures result in higher-energy configurations being involved, possibly with infinite action. An elegant way to take into account such terms [21] suggests to add so-called meron solutions. In fact, originally proposed in the framework of Yang–Mills theory [19] , the meron is characterized by a non-integer topological charge, namely 1/2. In this spirit, a finite-action solution with topological charge 1 can be made of two merons with finite separation (a bound meron pair) that breaks up into constituents when large distance effects become prominent. Hereafter, the terms half-skyrmion or meron and half-antiskyrmion or antimeron will be considered as synonymous. In general, a skyrmion that moves towards an edge becomes annihilated. However, for the kagome magnet the annihilation of the skyrmion does not occur once it reaches the edge, since the existence of chiral magnonic edge states gives rise to profound changes in the excitations of the kagome lattice, as we have seen in Fig. 2 . Thus, once the SA pair reaches the edge, the chirality forces them to be separated as two distinct entities. As shown in Fig. 3a , the meron and antimeron emanating from the collision of the SA pair at the edge of the kagome lattice have drastically different speeds, since the distance travelled by the antimeron is shorter than the one of the meron during the same period of time. A magnification of the SA pair discussed in Fig. 3a is shown in Fig. 4 . For further discussions about the connection between speed and the strength of interaction parameters of the Hamiltonian, see Supplementary Note 5 . Notice that because of the chosen magnetic orientation of the spins studied here, the meron has counterclockwise chirality contrary to the antimeron, which has clockwise chirality. In Fig. 4a we show the coupled SA pair, just before it reaches the edge. Note that the dashed line shows the magnetic texture for a half-antiskyrmion. Hence, this illustrates how the SA pair is coupled before it reaches the edge. 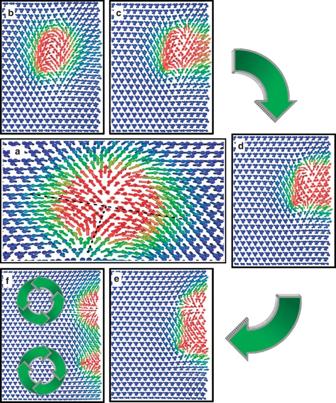Figure 4: Snapshots of a coupled skyrmion–antiskyrmion pair colliding with the edge of the kagome stripe. (a) Illustration of a skyrmion–antiskyrmion pair before the collision with the edge of the kagome stripe. Dashed lines are a guide to the eye for recognizing the antiskyrmion magnetic texture, while the other half of the magnetic excitation resembles a magnetic texture like in the Belavin–Polyakov monopole. (b–f) Several frames showing the coupled SA pair colliding with the edge of the stripe and the resulting SA decoupling because of the chiral edge states. The snapshots were taken from the same simulation displayed inFig. 3a. Figure 4b–f shows the time evolution of this SA pair over a time interval of 90 ps, just before ( Fig. 4b ) and just after ( Fig. 4c–f ) it reaches the edge. Note that once the coupled SA pair reaches the edge, it becomes unstable, due to non-trivial topology, and breaks up into a separated meron and antimeron ( Fig. 4e,f ), and then they travel along the edge in a decoupled manner with opposite directions. Figure 4: Snapshots of a coupled skyrmion–antiskyrmion pair colliding with the edge of the kagome stripe. ( a ) Illustration of a skyrmion–antiskyrmion pair before the collision with the edge of the kagome stripe. Dashed lines are a guide to the eye for recognizing the antiskyrmion magnetic texture, while the other half of the magnetic excitation resembles a magnetic texture like in the Belavin–Polyakov monopole. ( b – f ) Several frames showing the coupled SA pair colliding with the edge of the stripe and the resulting SA decoupling because of the chiral edge states. The snapshots were taken from the same simulation displayed in Fig. 3a . Full size image The results of Figs 3 and 4 demonstrate that it is possible to create SA pairs in a kagome lattice and that they are stable over a substantial period of time. It is also clear that SA pairs can travel with supersonic velocities of ~1,300 m s −1 . However, the linear momentum of such SA pairs is unfortunately difficult to control or design by the initial conditions of their generation. A way to overcome this problem is to make use of the topological properties of the edge states of the kagome magnet and to place the local excitation at the edge of the sample. In Fig. 5 and in Supplementary Movies 3 and 4 , we illustrate as an example the generation and time evolution of a skyrmion and antiskyrmion pair, created in exactly the same way as described in Fig. 3 . In Fig. 5a it is shown that the meron moves to the right side, whereas the antimeron travels in the opposite direction. The difference in their direction is produced by their different chirality (see Supplementary Note 1 ). Local excitations placed at the edge do not always generate SA pairs; it is quite possible that single merons are generated. As an example we show in Fig. 5b a singular meron (the antimeron is indeed created also here but is damped out very quickly). 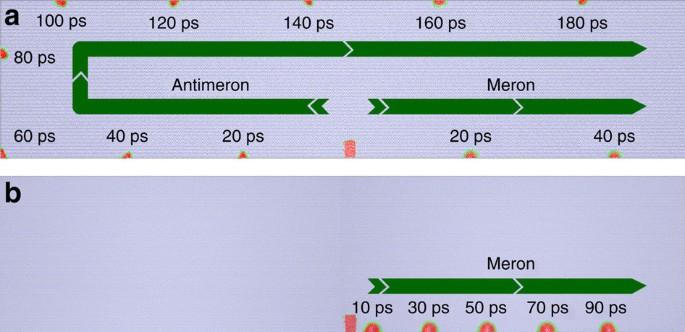Figure 5: Snapshots of skyrmionic excitations at the edge of the kagome stripe. (a) Generation and stabilization of a meron and an antimeron. In this case, the antimeron is able to overcome a 90 degree bend (Supplementary Movie 3). (b) Generation and time evolution of a single meron. The antimeron is damped out very quickly after it is generated (Supplementary Movie 4). In both cases (a,b), the meron moves counterclokwise and the antimeron clockwise. In both figures, the calculations were performed withT=1 mK,mRy andmRy. Figure 5: Snapshots of skyrmionic excitations at the edge of the kagome stripe. ( a ) Generation and stabilization of a meron and an antimeron. In this case, the antimeron is able to overcome a 90 degree bend ( Supplementary Movie 3 ). ( b ) Generation and time evolution of a single meron. The antimeron is damped out very quickly after it is generated ( Supplementary Movie 4 ). In both cases ( a , b ), the meron moves counterclokwise and the antimeron clockwise. In both figures, the calculations were performed with T =1 mK, mRy and mRy. Full size image The important message from the results of Fig. 5 is that the direction of the meron and antimeron is totally controlled at the edge of the kagome lattice. Indeed, the topological nature of these excitations prevents the meron or antimeron to leave the edge, or to collapse. The stability of these chiral excitations is illustrated further by the fact that they can survive travelling along a 90 degree corner, as is shown in Fig. 5a and Supplementary Movie 3 , for an antimeron. The strong stability and long lifetimes of these excitations become promising when considering applications because magnetic information can be transported over long distances along complicated paths and for long times. Our results suggest that it is quite possible to create a meron (write) at one point of space and time and to detected it (read) at another distant point along the edge. This property paves the way for novel applications of skyrmions similar to, for example, performing logical operations (skyrmionics). Collision of topological excitations Our results so far point out that it is possible to create skyrmionic excitations that can move with significant speed along edges and it is natural to ask whether collisions between such particle-like excitations can happen, and if so, how do they happen? To unravel this question, we have studied meron–meron and meron–antimeron collisions (at T =1 mK). This was performed by creating, simultaneously, two excitations at the edge of the kagome lattice. The excitations were created with sufficient distance, in order to avoid any initial interaction or correlation between them because of the emission of short lifetime spin waves generated during the excitation of the system. Once the two edge skyrmions were excited they started to travel counterclockwise along the edge of the lattice, the first (meron a ) being ahead of the second (meron b ). For this particular pair of merons, the second one had higher speed, hence allowing for investigating a meron–meron collision. In Fig. 6 , three snapshots show the moment before ( t 0 ), during ( t 1 ) and after ( t 2 ) this collision. As the figure and Supplementary Movie 5 shows, the two merons seems to experience an elastic collision, so that before the collision ( t 0 ) meron b has a linear momentum that is larger than that of meron a . At the collision ( t 1 ), the meron b provides linear momentum to meron a , in such a way that 10 ps after the collision ( t 2 ), meron a has a higher momentum than meron b . 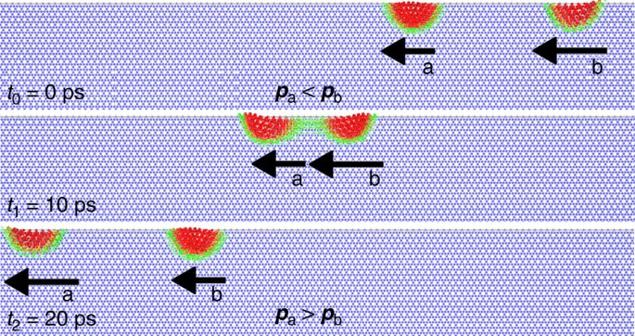Figure 6: Snapshots of the meron–meron collision. Att0, meronbhas higher linear momentum (pb) than merona(pa) but 10 ps after the collision (t2), meronamoves away from meronbwith higher velocity (Supplementary Movie 5). The simulations were performed atT=1 mK,mRy andmRy. Figure 6: Snapshots of the meron–meron collision. At t 0 , meron b has higher linear momentum ( p b ) than meron a ( p a ) but 10 ps after the collision ( t 2 ), meron a moves away from meron b with higher velocity ( Supplementary Movie 5 ). The simulations were performed at T =1 mK, mRy and mRy. Full size image The results of Fig. 6 pose questions regarding the details of a seemingly elastic collision. We analyse this by considering that the dynamics of the meron travelling along the x direction can be described by the Lagrangian , where x is the coordinate of the meron centre of mass and m is the ‘mass’ of the meron. The ‘mass’ is considered to be equal to the number of spins constituting the meron and the momentum is then . It should be noted that it is not possible to exactly specify the boundary of a meron because of the discrete nature of the spin lattice. Hence, the calculation of the ‘mass’ of a meron is associated with a small numerical error. Nevertheless, the calculated masses for the merons in Fig. 6 , before the collision, are m a ≃ 176 spins and m b ≃ 210 spins, while after the collision, they change the mass slightly, becoming m a ≃ 220 spins and m b ≃ 182 spins. We have also evaluated the velocities of the merons just before and after the collision and hence been able to analyse the linear momentum of the collision in Fig. 6 . The total linear momentum before the collision is about P x ≃ 4,652 (Å spins) per ps and after the collision it is P x ≃ 4,620 (Å spins) per ps. Moreover, we have also computed the kinetic energy before and after the collision and found that it is 11.40 and 11.30 (Å ps −1 ) 2 spin, respectively. Hence, within numerical errors, both the linear momentum and kinetic energy are conserved, demonstrating the elastic nature of the collision in Fig. 6 . In contrast to elastic collisions of purely classical systems the mass of an individual meron is not conserved during the collision in Fig. 6 . It is also possible to investigate meron–antimeron collisions and we show in Fig. 7 several snapshots of the generation of a meron and an antimeron and their time evolution. 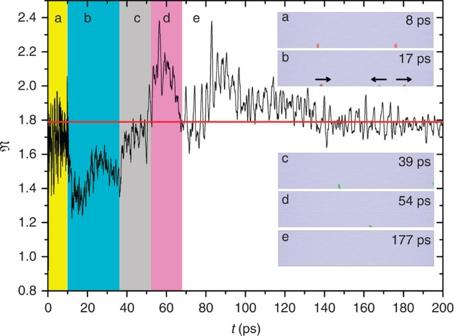Figure 7: Snapshots at different stages of the meron–antimeron annihilation process. (a) Two red regions at the lower edge of the kagome stripe are shown in the figure with reversed magnetization, due to a local applied torque. (b) Generation of two merons and one antimeron after removing the local torque from the surface. (c) Meron–antimeron annihilation collision. (d) Generation of a second meron as a result of the emission of spin waves in the annihilation collision observed in (c). (e) Equilibration of the spin waves. The figure also illustrates the time dependence of the total skyrmion number. The horizontal red line indicates the skyrmion number at the first time step (Supplementary Movie 6). Here the calculations were performed at T=1 mK,mRy andmRy. Figure 7 and Supplementary Movie 6 show that once created, they move towards each other. Figure 7 also shows the time evolution of the skyrmion number of the whole simulation cell. The skyrmion number was calculated as shown in the Methods section at every simulation time step. Similar to the generation of the separated pair of skyrmionic excitations ( Fig. 6 ), the skyrmion–antiskyrmion pair was generated at the edge, by first reversing moments in a region by a local torque and then (after 10 ps) removing this torque rapidly. Looking at the details of Fig. 7 , we note that initially a meron–antimeron is generated at the right hand side of the sample and only a single meron is generated on the left side. We hence have three dynamical excitations that we will refer to as the right meron (from the right side of the sample), the left meron (from the left side of the sample) and the antimeron. Figure 7 shows that the right meron gets damped after a while and leaves the system. The left meron and the antimeron are more long-lived and are found to move towards each other and collide after 39 ps ( Fig. 7c ). At this collision, they fuse and destroy each other. As a result, the energy is carried out by outgoing spin waves, which after 54 ps create a meron in a totally different part of the lattice ( Fig. 7d ) that subsequently moves to the right along the edge before it gets damped and leaves the system. The spin dynamics hence shows a very non-localized process of the destruction and creation of skyrmionic excitations. Figure 7: Snapshots at different stages of the meron–antimeron annihilation process. ( a ) Two red regions at the lower edge of the kagome stripe are shown in the figure with reversed magnetization, due to a local applied torque. ( b ) Generation of two merons and one antimeron after removing the local torque from the surface. ( c ) Meron–antimeron annihilation collision. ( d ) Generation of a second meron as a result of the emission of spin waves in the annihilation collision observed in ( c ). ( e ) Equilibration of the spin waves. The figure also illustrates the time dependence of the total skyrmion number . The horizontal red line indicates the skyrmion number at the first time step ( Supplementary Movie 6 ). Here the calculations were performed at T=1 mK, mRy and mRy. Full size image Figure 7 also shows that the skyrmion number ( ) is not an integer and it is not very smooth as a function of time. This behaviour is because of the fact that the skyrmion number was calculated for the whole sample and we used a very low damping. In consequence, there are contributions to arising also from regions far away from the place where the skyrmionic excitations are located. We can nevertheless get some insight from this number if we concentrate on the difference of this parameter at certain time steps. The horizontal red line indicates the value of the skyrmion number for the initial step; therefore, we take this value as the background skyrmion number. During the first 10 ps (yellow region), the applied local torques are present. In region b, just after the creation of the topological excitations, the skyrmion number is reduced with roughly 0.5. This is because we have created an antimeron with skyrmion number −0.5. In the transition b→c, the meron–antimeron collision is produced and they annihilate each other while the remaining meron shown on the right side dies after colliding with the vertical edge. In region c, the skyrmion number tends to come back towards the ground value with a jump of ~0.5 because the antimeron was annihilated. In this region we still can appreciate the remaining meron just before dying. In region d, the increase in the skyrmion number of ~0.5 is because of the creation of another meron. This excitation is created by spin waves that were emitted during the meron–antimeron annihilation. This object is however damped away very quickly with strong spin wave activity during the first part of region e. After some time, the system equilibrates and the skyrmion number goes back to the initial value as it is observed in Fig. 7e . Topological excitations at room temperature Recent experimental results on chiral bulk magnets such as MnSi (ref. 22 ) and Fe 0.5 Co 0.5 Si (ref. 23 ) have indeed identified a skyrmion lattice phase. These works came to the conclusion that the so-called skyrmionic ‘A phase’ is stabilized in a very limited region of a phase diagram defined by the applied magnetic field and temperature of the sample. The onset of the skyrmionic ‘A phase’ is observed only in a narrow window of this phase diagram, at around B =20 mT and T =25–30 K. Spin-polarized scanning tunnelling experiments of Fe monolayers (MLs) grown on Ir(111) also show that skyrmions are observed only at very low temperatures ( T =11 K) [24] . As far as we know, the highest temperature for the skyrmionic phase has been reported in ref. 25 , where the skyrmions have been manipulated with electrical currents at temperatures up to 275 K in FeGe. All in all, this makes these excitations less suitable for room temperature applications. However, our theoretical considerations outlined above show that SA pairs and merons generated in a kagome lattice do not have this limitation. As an example, we show in Fig. 8 and Supplementary Movies 7 and 8 , the generation and movement of bulk and edge skyrmions at a temperature of 300 K. In this section, we discuss about general conditions for the stabilization of topological excitations at room temperature, so that the model parameters are not related to a specific material. 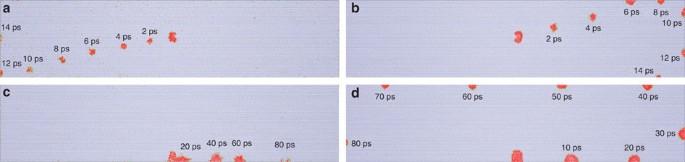Figure 8: Snapshots of skyrmionic excitations at room temperature. Panel (a) shows the creation of an SA pair and (c) an edge meron, usingmRy andmRy (Supplementary Movie 7). Inbwe show an SA pair and indan edge meron, usingmRy andmRy (Supplementary Movie 8). Figure 8a,b shows the creation and temporal evolution of bulk skyrmions, whereas Fig. 8c,d shows edge skyrmions. Note that the strength of the exchange and DM interaction in Fig. 8b,d is twice as large as that used in Fig. 8a,c . Figure 8: Snapshots of skyrmionic excitations at room temperature. Panel ( a ) shows the creation of an SA pair and ( c ) an edge meron, using mRy and mRy ( Supplementary Movie 7 ). In b we show an SA pair and in d an edge meron, using mRy and mRy ( Supplementary Movie 8 ). Full size image As regards suitable materials for which the here-predicted phenomena should be possible to observe at room temperature, we note that larger values of and have a better chance for stabilizing skyrmions. However, the skyrmionic excitations discussed here are stable for a wide range of and . Thus, for example, for the exchange interaction was ranged from 1 to 10 mRy in steps of 1 mRy, while was varied from 0.4 to 4 mRy in steps of 0.4 mRy. Skyrmionic excitations become to be more stable when mRy and mRy (for example, as shown in Fig. 8 ). For cases in which mRy, skyrmions are still visible but their shape is not well defined and skyrmionic excitations with lower values of and have higher probability to be damped away just after their creation. As shown in Fig. 8b,d , larger values of and results in skyrmions that are more stable and less susceptible from thermal fluctuations. Simulations for different ratios between the strength of the exchange and DM interaction were performed and the results clearly show that the ratio influences the stability of skyrmionic excitations. Thus, as an example, for and 0.2 both merons and SA pairs are unstable in the range of 1–10 mRy, while for topological excitations stabilize at and for the meron becomes stable for . The criterion for the stabilization is associated here with the total simulation time, so that the skyrmionic excitations are considered as stable if they overcome the threshold of 100 ps. There are several materials for which the exchange interaction is either measured experimentally or calculated from first principles to lie in the range of energies we have used in the present simulations. The challenge is to tune the DM interaction. Figure 8a shows room temperature skyrmions for a calculation with a DM interaction with strength of 2 mRy. This is actually not too different from the DM interaction of some thin film systems, for example, two MLs of Fe on W (110). In this system, a spin wave asymmetry of 12 meV was calculated from first principles [26] . In addition, it should be noted that the thermal stability is enhanced for a given set of parameters of the Hamiltonian, when considering more than one layer of the kagome lattice. For instance, we have performed several simulations varying the number of layers, for example, two and four MLs. In these simulations, we considered as intralayer parameters mRy and mRy (that is, a lower DM interaction than that the one reported in ref. 26 ) and as interlayer parameters mRy and mRy, and we estimated the Curie temperature from mean-field theory. For two MLs, we have found T c =372 K, while for four MLs we found T c =419 K. The main message of these simulations is that the number of magnetic layers is an important parameter that enhances the Curie temperature, and therefore, it is possible to deal with very realistic parameters to achieve room temperature skyrmions. In addition to thin film systems, we observe that bulk materials can also play an important role for stabilizing skyrmions at room temperature. We suggest that Fe 3 Sn 2 is such a material [27] . In this material, Fe ions form bilayers of offset kagome networks, while the Sn ions occupy two distinct crystallographic sites. Thus, Sn ions lie within the kagome layers as well as between the kagome bilayers. An important characteristic of this material is that the T c is ~640 K, and that there are experimental observations that suggest that after the ferromagnetic phase is stabilized at 640 K, upon further cooling non-trivial magnetic phases are formed. A further investigation of this material is outside the scope of the present paper; however, we point out that in both thin film and bulk materials there is a chance to observe room temperature skyrmions. We have outlined conditions for novel exotic magnetic excitations of the kagome lattice. The possibility to observe bulk and edge states is outlined here, where, in particular, the edge states have non-trivial topological properties that provide unique magnon modes. We have also shown that the kagome lattice has potential to exhibit SA pairs, meron and antimeron excitations even at room temperature. This is found for a wide range of parameters describing the magnetic excitations, in particular, the DM interaction and the Heisenberg exchange interaction. It is important to notice that the effective 2D kagome lattice has the DM interaction merely confined within the 2D plane; however, there are still interlayer exchange interactions that can affect the behaviour of the reported topological excitations and their collisions. In order to deal with this issue, we performed simulations with several stacked layers of 2D kagome planes coupled by an exchange interaction of 1 mRy. The results show that the interlayer exchange interaction does not affect the stability of the skyrmionic excitations (see Supplementary Note 6 and Supplementary Movie 9 for further details). Owing to the non-trivial topology of the edge states, we find that it is possible to control the movement of skyrmionic excitations and that such excitations are long-lived. We have even found that these particle-like excitations can move on well-defined straight lines and even be made to turn around corners. This offers a potential to use such excitations in different emerging technologies such as, for example, in data storage or manipulation of magnetic bits. We have also investigated meron–meron and meron–antimeron collisions. The former are found to undergo elastic collisions, whereas the latter are more complex. Thus, the annihilation of a meron–antimeron collision is followed by the creation of a new meron, a process which occurs as a highly non-local phenomenon. Pyrochlores are possible candidates for observing the phenomena predicted in this work and particularly we discussed here the 111-cut of the vanadate pyrochlores. The kagome lattice can, however, be found in many other compounds, for example, SrCr 8 Ga 4 O 19 (ref. 28 ), Ba 2 Sn 2 Ga 3 ZnCr 7 O 22 (ref. 29 ) and the jarosites like KM 3 (OH) 6 (SO 4 ) 2 (refs 30 , 31 , 32 ) with M=V, Cr or Fe. These materials are also potential candidates for investigations of non-trivial topological magnon edge states and skyrmionic excitations at very low temperature. Model hamiltonian Our theoretical methodology [33] consists of mapping an itinerant electron system on an effective spin-Hamiltonian [34] , [35] , where < ij > denotes the atomic indices to the first neighbour pairs, s i is the atomic moment, is the strength of the exchange interaction and the SO contribution is included via the strength of the DM vector . The last term comes from the Zeeman effect under an external magnetic field B , where g is the g-factor and μ B represents the Bohr magneton. We consider that the exchange interaction as well as the modulus of the DM vector are the same for every pair of atoms, which is consistent with all atoms of the kagome lattice being of the same type. Hence, we use and . Atomistic spin dynamics In order to capture the dynamical properties of spin systems at finite temperatures we used an atomistic spin dynamics (ASD) approach [33] . The equation of motion of the classical atomistic spins at finite temperature is governed by Langevin dynamics via a stochastic differential equation, normally referred to as the atomistic Landau–Lifshitz–Gilbert equations, which can be written in the form: where γ is the gyromagnetic ratio and α i denotes a dimensionless site-resolved damping parameter that accounts for the energy dissipation that eventually brings the system into a thermal equilibrium. The effective field in this equation is calculated as and the temperature fluctuations ( T ) are considered through a random Gaussian shaped field b i ( t ) with the following stochastic properties: where i and j are atomic sites, while μ and ν represent cartesian coordinates of the stochastic field. After solving the Landau–Lifshitz–Gilbert equations, we have direct access to the dynamics of the atomic magnetic moments s i ( t ) and with this information we can calculate all relevant dynamical properties such as the connected space- and time-displaced correlation functions defined as where ‹ ⋯ › denotes an ensemble average and k is the cartesian component. The magnon dispersion relation can be evaluated via the dynamic structure factor S ( q , ω ), which is nothing else than the space and time Fourier transform of the connected correlation function, where N is the number of terms in the summation, while q and ω are the momentum and energy transfer, respectively (see Supplementary Note 4 for further details about the simulations). Pontryagin index The skyrmion number or Pontryagin index represents a topological index of the field configuration and is defined and evaluated here, by where represents a 2D compact orientable manifold. The topological excitation with is called a skyrmion, while in the case of it is termed an antiskyrmion. The same formalism can be extended straightforwardly to describe multiskyrmionic states and in particular skyrmion–antiskyrmion pairs [36] . How to cite this article: Pereiro, M. et al. Topological excitations in a kagome magnet. Nat. Commun. 5:4815 doi: 10.1038/ncomms5815 (2014).